Colossal positive and negative thermal expansion and thermosalient effect in a pentamorphic organometallic martensite The thermosalient effect is an extremely rare propensity of certain crystalline solids for self-actuation by elastic deformation or by a ballistic event. Here we present direct evidence for the driving force behind this impressive crystal motility. Crystals of a prototypical thermosalient material, (phenylazophenyl)palladium hexafluoroacetylacetonate, can switch between five crystal structures (α—ε) that are related by four phase transitions including one thermosalient transition (α↔γ). The mechanical effect is driven by a uniaxial negative expansion that is compensated by unusually large positive axial expansion (260 × 10 –6 K –1 ) with volumetric expansion coefficients (≈250 × 10 –6 K –1 ) that are among the highest values reported in molecular solids thus far. The habit plane advances at ~10 4 times the rate observed with non-thermosalient transitions. This rapid expansion of the crystal following the phase switching is the driving force for occurrence of the thermosalient effect. Biogenic mechanical processes in living organisms present important mechanistic and kinematic models for the design of biomimetic actuators [1] , [2] , [3] . The capability of rapid energy transfer through the dense and ordered packing of molecular single crystals evolves as a new platform for efficient actuation. Dynamic single crystals capable of bending, twisting, curling, rolling or locomotion [4] , [5] , [6] , [7] , [8] , [9] , [10] are prospective candidates for the design of dynamic elements, including artificial tissues and components in microfluidic devices. The fast energy transfer secured by efficient coupling between the thermal/light energy and mechanical energy stands as their main asset towards the design of fast actuators. Performance optimization of such technomimetic and biomimetic single crystals necessitates understanding of the underlying atomic-scale processes. Anomalous cell expansion in some of these materials, such as unusually large positive thermal expansion (PTE) and negative thermal expansion (NTE), adds a special interest in their structural science [11] , [12] , [13] , [14] , [15] , [16] . In a short article from 1983, Etter and Siedle [17] briefly noted that when yellow crystals of (phenylazophenyl)palladium hexafluoroacetylacetonate (PHA) are heated on one side ‘[the crystals] literally fly off the hot stage’. This observation of crystal motility was to become the first documented report of the thermosalient (TS) effect (Hüpf-Effekt)—the propensity of certain crystals to hop and leap when heated over a phase transition [9] , [10] , [18] , [19] . Two polymorphs, yellow form (α) and red form (β), were characterized [17] . Although this material could provide direct insight into the response of ordered matter to extreme internal pressures, the relationships between the structural, mechanistic and kinematic aspects of the TS effect remain poorly understood. To decipher the interplay between the thermodynamic and kinetic profile of the TS effect, we investigated the mechanistic aspects of the motility of PHA crystals as a prototypic TS structure where (in contrast with other TS solids) during the leaping the macroscopic integrity of the crystals is preserved. Additional motivation for this study was a video recording of Etter’s [17] last lecture from 1992 (retrieved by a kind courtesy of Joel Bernstein from his private collection), where she mentions that conversion between the yellow phase α and the red phase β underlying the crystal hopping proceeds through an intermediate ‘expanded yellow form’. The crystal structure of the ‘expanded yellow form’, and thus the mechanism of the actuation, has not been resolved before this study. The results presented herein unravel the extraordinary complex crystal chemistry of PHA, which also sets the record for the largest number of polymorphs of an organometallic material. We report three new polymorphs: form γ, which is a product of the transition that drives the TS effect, as well as two low-temperature (LT) forms (δ and ε). At least two forms undergo exceptionally large PTE. With one of the polymorphs, which also undergoes uniaxial NTE, we measure some of the largest thermal expansion coefficients ever reported. We also establish a direct link between the anomalous thermal expansion and the mechanical response, both phenomena being rooted in the susceptibility of this structure to internal strain. TS effect in PHA Crystals of the two polymorphs of PHA, prepared according to a previously published procedure [20] , were obtained by recrystallization or sublimation ( Supplementary Fig. 1 ) and identified by X-ray diffraction (XRD) as the yellow (α) and red (β) forms described by Etter and Siedle [17] . The thermal behaviour of the two polymorphs was monitored by differential scanning calorimetry (DSC) and hot-stage microscopy. While heating up to the decomposition temperature did not have any effect on the crystals of form β, when heated over 343 K crystals of form α responded with forceful jumps ( Supplementary Movie 1 ). To understand the kinematic details of this mechanical effect, the trajectories of 95 heated crystals of form α were analysed from high-speed digital recordings (resolution: 10 3 s –1 ) and batched according to their kinematic effect and metrics (to account for the different number of crystals in each group, the number of crystals that underwent certain effect was normalized against the total number of crystals in the batch). The kinematic analysis showed that the crystal motility occurs as two kinematic effects ( Fig. 1a,b and Supplementary Movies 2–5 ): expansion (effect 1 ) and expansion followed by hopping (effect 2 ), whereby crystals hop off the surface to flip several times before landing. The number of crystals that expand (effect 1 ) increases with their length ( Fig. 1c–f ) [21] . 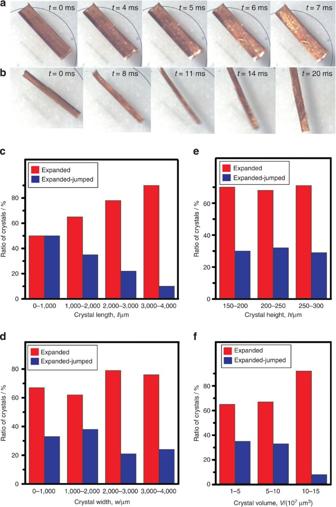Figure 1: The TS effect in crystals of PHA. (a,b) Snapshots, taken at frequency 103s–1, of the two kinematic effects, expansion (effect1) and expansion followed by hopping of the crystals off the base (effect2). (c–f) Distribution of the relative ratio of the two kinematic effects of PHA crystals over the crystal metrics. To account for the natural distribution of crystal size, the number of crystals undergoing particular effect in each batch was divided by the total number of crystals in the same batch. Figure 1: The TS effect in crystals of PHA. ( a , b ) Snapshots, taken at frequency 10 3 s –1 , of the two kinematic effects, expansion (effect 1 ) and expansion followed by hopping of the crystals off the base (effect 2 ). ( c – f ) Distribution of the relative ratio of the two kinematic effects of PHA crystals over the crystal metrics. To account for the natural distribution of crystal size, the number of crystals undergoing particular effect in each batch was divided by the total number of crystals in the same batch. Full size image High-temperature phase transitions Hot-stage microscopy ( Supplementary Fig. 2 ) indicated that when heated above room temperature (RT) crystals of form α did not transform to form β directly. When a yellow crystal of form α was heated with a stream of nitrogen gas, it initially underwent gradual colour change from yellow to orange-yellow ( Fig. 2a ). Around 347 K (uncorrected value), the crystal suddenly expanded along (100) and turned dark orange, but remained clear and transparent. In case of thick pristine crystals, the expansion was occasionally accompanied by splitting parallel to the longest axis. The DSC curve of this first stage displays a series of sharp endothermic peaks between 342.7 and 354.5 K ( Fig. 2f ). Temperature- and time-resolved in situ X-ray powder diffraction (XRPD; Supplementary Fig. 7 ) analysis confirmed that in the bulk the new phase, form γ, coexisted with forms α and β. 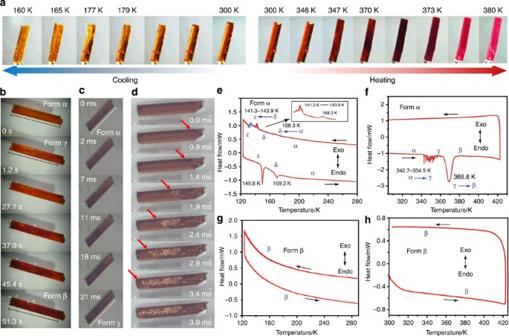Figure 2: Crystal habit and thermochromic and thermal profile of PHA crystals. (a) Morphology and colour of single crystals of PHA that were cooled and heated in a stream of nitrogen gas (the temperature values are uncorrected). Note the expansion of the crystal at HT and the splitting into fibrous microcrystals at LT. The overall brightness of the photographs was enhanced uniformly for clarity. (b–d). High-speed snapshots of the migration of the habit plane and colour change during the phase transition. The edge of the habit plane is marked with red arrow ind. (e–h) Heat effects and phase transitions upon thermal cycling of PHA monitored by DSC (heating/cooling rate: 10 K min–1). Figure 2: Crystal habit and thermochromic and thermal profile of PHA crystals. ( a ) Morphology and colour of single crystals of PHA that were cooled and heated in a stream of nitrogen gas (the temperature values are uncorrected). Note the expansion of the crystal at HT and the splitting into fibrous microcrystals at LT. The overall brightness of the photographs was enhanced uniformly for clarity. ( b – d ). High-speed snapshots of the migration of the habit plane and colour change during the phase transition. The edge of the habit plane is marked with red arrow in d . ( e – h ) Heat effects and phase transitions upon thermal cycling of PHA monitored by DSC (heating/cooling rate: 10 K min –1 ). Full size image The first-order transition α→γ is reversible, and if the crystal is not heated to higher temperature form α can be recovered from form γ by cooling. Upon further heating, however, the elongated orange crystals of the in situ generated form γ underwent a second transition at 367.4 K (DSC) without visible changes in size and morphology, whereupon they slowly and gradually turned dark red and became opaque ( Fig. 2a , and Supplementary Fig. 2 and Movie 6 ). The phase transition γ→β was not mechanically active and the crystals remained still. This transition is irreversible; no thermal effects were observed for form β (obtained either by heating of form α or by crystallization) between 120 and 430 K ( Figs 2g,h and 3b , and Supplementary Fig. 5 ), indicating a thermodynamically stable structure. 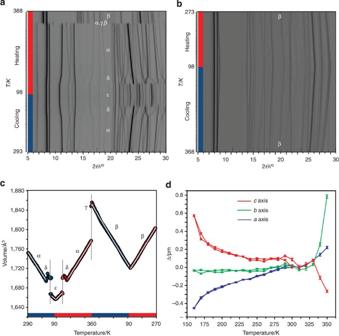Figure 3: Phase transitions of PHA and unit cell deformation. (a,b) Phase transitions of polymorphs α and β monitored by temperature-resolved XRPD. (c) Change of the unit cell volume with temperature based on XRPD data (the volumes of forms γ and β were doubled to bring them on the same scale as the data for α); and (d) temperature dependence of the unit cell parameters of form α extracted from single-crystal XRD data relative to their values at 300 K. The error bars represent the respective s.d. Figure 3: Phase transitions of PHA and unit cell deformation. ( a , b ) Phase transitions of polymorphs α and β monitored by temperature-resolved XRPD. ( c ) Change of the unit cell volume with temperature based on XRPD data (the volumes of forms γ and β were doubled to bring them on the same scale as the data for α); and ( d ) temperature dependence of the unit cell parameters of form α extracted from single-crystal XRD data relative to their values at 300 K. The error bars represent the respective s.d. Full size image Although the generation of form γ was clearly confirmed by DSC, optical/Raman microscopy ( Supplementary Fig. 6 ) and XRPD ( Fig. 3a,c , see also Supplementary Figs 7 and 8 ), because of the very narrow thermal stability window and the dependence of the transition temperature on crystallite size and shear history (see below), we could only obtain bulk amounts of form γ as a ternary mixture with forms α and β ( Fig. 3a ). We monitored the high-temperature (HT) transitions with in situ XRPD ( Supplementary Figs 7 and 8 ). Rietveld refinement of the mixture confirmed that form γ was produced in 54.63% yield, and coexisted with form β (39.56%) and a small amount (5.80%) of untransformed form α ( Supplementary Fig. 9 ). The gratifying occurrence of both TS and non-TS phase transitions of PHA and the crystal structures of forms α, β and γ set the basis to establish the molecular mechanism of the TS effect ( Fig. 4 and Supplementary Fig. 19 ). The structure of α is composed of layers of head-to-head slip-stack molecules ( Fig. 5 ). At RT, the molecules of the adjacent layers are at distances d (Pd···Pd) out-of-plane =3.7839(3) and 4.8166(3) Å (298 K; Supplementary Table 5 ). 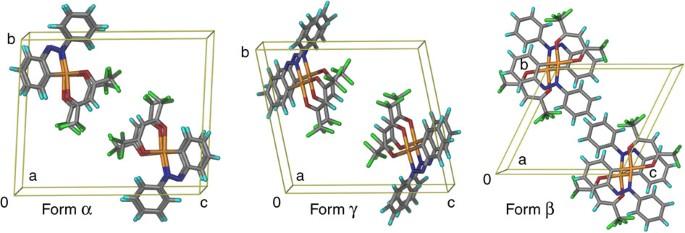Figure 5: Crystallographic relation between the three HT phases of PHA. The TS transition (from form α to γ) is related to separation of the head-to-head stacked molecules. During the non-TS transition (from form γ to β), the molecules from alternating layers slip in opposite directions resulting in interdigitated, head-to-tail-stacked layers. Form β is a thermodynamically stable polymorph and does not revert to any of the other forms by cooling (ambient pressure). By heating, the cell expands mainly along the a axis and the molecules are separated out to d (Pd···Pd) out-of-plane =3.8041(9) and 4.846(1) Å (320 K; Fig. 4 ). 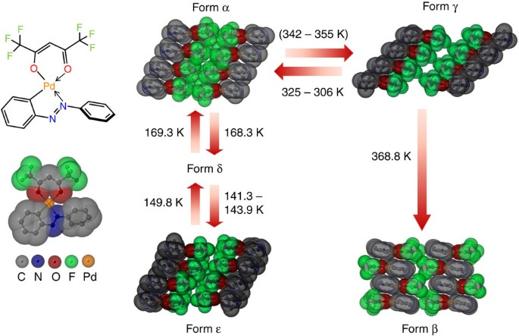The shear strain caused by the distortion of the unit cell accrues to the point where it overweighs the cohesive interactions, whereupon the packing of form α switches to that of form γ. Figure 4: Phase transitions and crystal structures of four of the five polymorphs of PHA. The crystal structures of forms α and β were determined from single crystals, and those of forms γ and ε were determined from powder diffraction data. During the TS transition (α→γ), the layers of molecules in form α slide atop each other, the columns of stacked molecules are slanted, and the adjacent molecules in head-to-head disposition are separated in form γ. γ is a metastable form, and in the second HT transition (γ→β) the alternating layers slide in opposite directions and interdigitate to a head-to-tail stacking pattern in the thermodynamically stable form β. The chemical structure of PHA and the colour-coding scheme used in the packing diagrams are shown on the left. Figure 4: Phase transitions and crystal structures of four of the five polymorphs of PHA. The crystal structures of forms α and β were determined from single crystals, and those of forms γ and ε were determined from powder diffraction data. During the TS transition (α→γ), the layers of molecules in form α slide atop each other, the columns of stacked molecules are slanted, and the adjacent molecules in head-to-head disposition are separated in form γ. γ is a metastable form, and in the second HT transition (γ→β) the alternating layers slide in opposite directions and interdigitate to a head-to-tail stacking pattern in the thermodynamically stable form β. The chemical structure of PHA and the colour-coding scheme used in the packing diagrams are shown on the left. Full size image Figure 5: Crystallographic relation between the three HT phases of PHA. The TS transition (from form α to γ) is related to separation of the head-to-head stacked molecules. During the non-TS transition (from form γ to β), the molecules from alternating layers slip in opposite directions resulting in interdigitated, head-to-tail-stacked layers. Form β is a thermodynamically stable polymorph and does not revert to any of the other forms by cooling (ambient pressure). Full size image The sustainability of the phase transition even under isothermal conditions that was apparent from the evolution of the XRPD pattern ( Supplementary Fig. 8 ), and was also as observed from the progression of the change throughout the crystal (see below), is an indication of strong coupling between the PHA molecules. As it is inferred from the normalized unit cell volume, the first-order TS phase transition α→γ is accompanied by strongly anisotropic expansion. A large portion of the interfacial strain that accumulates in the crystalline interior is rapidly converted into elastic energy required for crystal reconfiguration and kinetic energy of the propelled crystal. During the transition, the PHA molecules from adjacent layers are separated from a distance d (Pd···Pd) out-of-plane =3.8041(9) and 4.846(1) Å ( α , 320 K) to 4.274(3) Å ( γ , 358 K), however the head-to-head disposition within the layers is retained. Figure 5 represents the crystallographic relationship between the three HT phases. Unlike the transition α→γ, where the columnar stacks are strained and the molecules are separated from each other, the transition γ→β is related to drastic structural rearrangement where the head-to-head slip-stack molecules in form γ switch to head-to-tail in β. This molecular interdigitation is not readily explicable by separation of the stacks. Instead, by invoking the least-motion pathway for the γ→β transition, we envisage a mechanism where alternating layers of PHA molecules slide to opposite directions to achieve energetically stabilized head-to-tail stacking ( Fig. 4 ). This perturbation, which yields head-to-tail arrangement of PHA molecules that are spaced out at d (Pd···Pd) out-of-plane =3.4889(5) and 4.5062(6) Å in form β (298 K; Supplementary Table 5 ), is unsustainable and results in crystal fragmentation. Based on mechanistic considerations, we have suggested [10] that the saw-tooth DSC profile of TS effects is indicative of martensitic-type transitions [22] , however that hypothesis has not been substantiated experimentally yet. By using a high-speed camera operating at time-resolution of up to 10 4 s –1 , we monitored the real-time spatial progression of the habit plane (the dynamic interface between the two phases) during the α→γ transition in several PHA crystals that were restrained from hopping with a minimum amount of oil ( Fig. 2c,d , and Supplementary Movies 7 and 8 ). Thermal homogeneity of the heat bath was provided by the much smaller size of the crystals (<1 mm) relative to the uniformly heated area and the use of oil as heat-transfer medium for thermal equilibration (by using thermal camera, we confirmed that the spatial thermal gradient of the samples was <1 mK). The TS phase transition always started at the sharp terminus of the crystal and its front, which encloses an average angle of 37° with the edge of the crystal, advanced very rapidly parallel to the longest axis until the entire crystal has been converted ( Fig. 2c,d ). This angle corresponds to the angle between the PHA molecules and the a axis of form γ ( Supplementary Fig. 18 ). The progression of the habit plane vindicates activation of cooperative processes [23] , [24] . Taken together with the displacive, diffusionless transition with miniscule rearrangement incurred from the comparative analysis of the molecular packing in α and γ, this result strongly supports the view that the TS effect appears in effect of a transition similar to the martensitic transitions in inorganic materials. The rate of progression of the habit plane during the TS transition (approximated by linear growth and averaged over three crystals) was 0.54 m s –1 , which corresponds to a turnover number of 1.272 × 10 9 molecules per second ( Fig. 2d and Supplementary Tables 3 and 4 ). This propagation rate is four orders of magnitude faster than that of the second, non-TS transition (γ→β) where the habit plane moves at 4.34 × 10 –5 m s –1 and 1.026 × 10 5 molecules are converted per second ( Supplementary Movies 9 and 10 ). This rate also supersedes greatly the common spin-crossover (low spin–high spin) transitions, which occur on a time scale of 10 –5 m s –1 . Thus, the rapid spatial phase progression and the resulting sudden macroscopic expansion of the crystal are key driving factors for occurrence of the TS effect. On the contrary, as inspected by the development of the dark red colour, under identical conditions with those used for the TS transition α→γ, the non-TS transition γ→β starts at several nucleation sites simultaneously and slowly spreads radially. The nucleation sites that appeared at different points of the crystal interior could be related to defects created during the preceding transition α→γ. Thus, not only the rate but also the mechanisms of the two transitions are very different. During the experiments, we noted that application of shear stress had a profound effect on the phase equilibria of PHA. Manual grinding of the yellow phase α led to nearly complete suppression of the TS effect with extinction of the thermal signature of the α→γ transition ( Supplementary Fig. 3b ). We confirmed by XRPD that upon light grinding at RT PHA remains in form α, whereas upon coarse and prolonged grinding or by milling it is converted into form β ( Supplementary Fig. 10 ). When heated, only a portion of the ground form α converted to form γ; in many cases, form α converted directly to form β. The temperature of this transition was 373.4 K ( Supplementary Fig. 8a ). We conclude that soft and elastic packing is a prerequisite to accumulate sufficient stress required for the TS effect. These considerations are in line with the unusually high nanoelasticity that was recently observed with another TS solid, 1,2,4,5-tetrabromobenzene [21] . LT phase transitions While the thermodynamically stable form β did not exhibit any changes on cooling, crystals of form α continued to change their habit and cracked around 129 K ( Fig. 2a and Supplementary Fig. 2 ) as an indication of a phase transition at LT. On further cooling, the crystal suddenly split along the longest axis into a bunch of fine, long crystalline fibres, which is suggestive of a second phase transition at LT. The two LT phase transitions, α→δ at 168.3 K and δ→ε at 143.9–141.3 K, were confirmed by DSC ( Fig. 2e and Supplementary Fig. 4 ). These transitions are reversible, and on heating they occur at 149.8 K (ε→δ) and at 169.3 K (δ→α). As confirmed by in situ XRPD, in the bulk the two LT transitions occur at 173 K (α→δ) and at 133 K (δ→ε), and the reverse transitions occur at 143 K (ε→δ) and at 173 K (δ→α) ( Fig. 3c and Supplementary Fig. 11a ). These transitions are accompanied by negligible hysteresis Δ T =1.0 K in the case of the α↔δ transition and a wider hysteresis Δ T =5.9–8.5 K for the δ↔ε transition. At even lower temperatures, the transition δ↔ε occurred with sharp changes in lattice parameters. High-resolution synchrotron XRPD data of phase ε were collected and used to solve the crystal structure, and the model of the structure was confirmed by Rietveld refinement ( Supplementary Fig. 12 and Supplementary Table 1 ). The overall packing of ε resembles very closely that of form α; the PHA molecules, stacked face-to-face, are slightly bent and the slanted molecular columns are offset in respect to each other ( Fig. 4 ). Optical properties and electronic structure The colour of form α PHA crystals is orange-yellow at RT and reversibly changes to orange in form γ at HT, but turns to efflorescent yellow in forms δ and ε at LT ( Fig. 2a ). Temperature-induced colour change of a single polymorph whose structure has been determined at various temperatures could provide insight into whether the difference in colours between the polymorphs is due to molecular or to supramolecular factors. In the case of form α, although the main packing motive is retained, the d (Pd···Pd) out-of-plane distances in the LT and HT structures are considerably different (3.874(2)/4.31(2) Å and 3.8041(9)/4.846(1) Å at 150 and 320 K, respectively), as well as are the respective angles between the phenyl ring and the molecular plane (46.9/50.3° and 47.0/45.9°; for details, see Supplementary Table 1 ). When crystals of phases α and β are compared, the PHA molecules differ in the deflection angle of the phenyl ring; in form α the exo-phenyl ring is twisted more (47.2/46.0° at 298 K) than in form β (15.6° at 298 K). The origin of colour in PHA was assessed through the density functional theory (DFT)-modelled lowest transitions of a single PHA molecule ( Supplementary Figs 13–16 ). The HOMOs (highest occupied molecular orbitals) have essentially Pd d yz character along with a sizable contribution from the π orbitals of the azobenzene ligand. The HOMO-1 and HOMO-2 include contributions from d yz and d z 2 orbitals, respectively. The LUMOs (lowest unoccupied molecular orbitals) of both rotamers are dominated by the π * orbitals of the azobenzene ligand. A noteworthy inference from the electronic structure of PHA is the near degeneracy of the LUMOs in the two forms ( E LUMO (α)=−2.96 eV and E LUMO (β)=−3.02 eV) despite the greater stabilization of the HOMO of the ( in vacuo ) rotamer in α (0.09 eV) relative to β, leading to narrower HOMO–LUMO gap in the red isomer (β). Consequently, the low-energy transition bands in the red form ( λ max ≈454 nm) are red-shifted compared with the yellow form ( λ max ≈447 nm). Specifically, the calculated electronic spectrum of PHA in form α has its lowest energy bands at 446.9 nm ( f =0.0829) and 438.7 nm ( f =0.0300) that include major contributions from the HOMO→LUMO, HOMO-1→LUMO and HOMO-2→LUMO transitions ( Supplementary Table 2 ). These transitions are assigned to metal-to-ligand charge-transfer d → π * transitions and π → π * transitions of the ligand. In the structure of β, the lowest energy bands are red-shifted to 453.8 nm ( f =0.1603) and 446.0 nm ( f =0.0145), and include major contributions from the HOMO→LUMO, HOMO-1→LUMO, HOMO-2→LUMO and HOMO-3→LUMO transitions. Although the DFT results reproduce well the observed trends, they do not provide quantitative description, and thus intermolecular factors ought to be invoked to explain the strong colour change. The dark red colour of form β is due to a low-energy transition that extends to 600 nm. The small energy gap between the two rotamers in vacuo (0.68 kcal mol –1 ) discredits the ring rotation as main contributor to the spectral shifts ( Supplementary Fig. 17 ). Because intramolecular geometrical perturbations cannot account for this transition and this absorption does not have equivalent in the calculated spectra, we ascribe the colour change to progressively decreasing separation and weaker collective intermolecular electronic coupling between the coordination charge-transfer centres within the stacks. The colour change observed on cooling and heating of phase α appears to be in line with this scenario. The TS phase transition α→γ is related to offset of PHA molecules that decreases their overlap and exerts minor effect on the intermolecular electronic interactions; hence, the colour changes from yellow to dark orange. On the contrary, the non-TS transition γ→β is related to significant structural perturbation, whereas the vertical head-to-head packing is switched to head-to-tail. The change of molecular disposition exerts strong effect on the intermolecular interactions and results in drastic colour change from orange to dark red. The increased opacity by evolution of microfractures enhances this effect. Thermal expansion and contraction To unravel the thermal effects on the structure that drive the thermal transition, we studied the thermal expansion of the solid forms of PHA with variable-temperature XRPD ( Fig. 3 ). (The very narrow temperature range where form ε is stable restricted the data set to only 6 data points on cooling and 8 data points on heating.) The expansion of form α was monitored within its thermal stability window, that is, between the transitions α→δ (193 K on cooling) and α→γ (348 K on heating). As shown in Fig. 6 , between 223 and 348 K form α undergoes an exceedingly large PTE with linear expansion coefficient along the a axis α a =260.4(3) × 10 –6 K –1 . The expansion along the b axis α b =39.4(4) × 10 –6 K –1 is higher but comparable to values that are typically observed with molecular solids (0 × 10 –6 K –1 < α <20 × 10 –6 K –1 ) (ref. 11 ). The strong PTE along the a axis is compensated by a considerably large NTE along the c axis, with coefficient α c =–79.9(2) × 10 –6 K –1 . Although the biaxial PTE is partially compensated by uniaxial NTE, the volumetric thermal expansion is exceptionally large, α V =247.8(2) × 10 –6 K –1 . On the contrary, all axes of form β undergo positive expansion, having unusually large PTE coefficients, α a =124.0(2) × 10 –6 K –1 , α b =105.4(3) × 10 –6 K –1 and α c =114.9(3) × 10 –6 K –1 . The isotropic expansion of form β results in large volumetric expansion with α V =255.5(3) × 10 –6 K –1 , which, together with α, is among the largest values reported thus far. Indeed, the volumetric and some axial thermal expansion coefficients of the PHA polymorphs are higher than the coefficients that are deemed colossal, reported for Ag 3 [Co(CN) 6 ] ( α V =160 × 10 –6 K –1 , α a =150 × 10 –6 K –1 and α c =–130 × 10 –6 K –1 ) by Goodwin et al. [13] , [14] , and are comparable to those of a MOF (metal organic framework) material under vacuum ( α V =300 × 10 –6 K –1 , α a =230 × 10 –6 K –1 and α c =–170 × 10 –6 K –1 ) reported by Omary and colleagues [15] , and of ( S,S )-octa-3,5-diyn-2,7-diol ( α V =47–241 × 10 –6 K –1 , α a =515–156 × 10 –6 K –1 , α b =−85 to −63 × 10 –6 K –1 and α c =−204 to −45 × 10 –6 K –1 ) reported by Barbour and colleagues [16] . 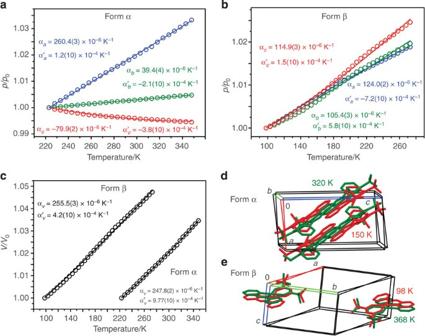Figure 6: Thermal expansion of PHA. (a) Biaxial PTE and uniaxial NTE of form α on heating from 223 to 348 K. (b) Axial PTE of β on heating from 98 to 273 K. (c) Volumetric PTE of forms α and β. (d) Crystal structures of form α at 150 K (red) and 320 K (green), and (e) of form β at 98 K (red) and 368 K (green) (Note that the unit cell of β is scaled to be comparable to the one of α.) The scattered data were collected from powdered samples and the lattice parameters were obtained by Pawley fitting of the diffraction patterns. The coefficients of thermal expansion were calculated using an expression having both linear and quadratic terms (the large uncertainty of the quadratic term, as well as visual inspection, indicates that the expansion is predominantly linear)p(T)=p0(1+αp(T–T0)(1+α′p(T–T0))) (ref.12). Figure 6: Thermal expansion of PHA. ( a ) Biaxial PTE and uniaxial NTE of form α on heating from 223 to 348 K. ( b ) Axial PTE of β on heating from 98 to 273 K. ( c ) Volumetric PTE of forms α and β. ( d ) Crystal structures of form α at 150 K (red) and 320 K (green), and ( e ) of form β at 98 K (red) and 368 K (green) (Note that the unit cell of β is scaled to be comparable to the one of α.) The scattered data were collected from powdered samples and the lattice parameters were obtained by Pawley fitting of the diffraction patterns. The coefficients of thermal expansion were calculated using an expression having both linear and quadratic terms (the large uncertainty of the quadratic term, as well as visual inspection, indicates that the expansion is predominantly linear) p ( T )= p 0 (1+ α p ( T – T 0 )(1+ α ′ p ( T – T 0 ))) (ref. 12 ). Full size image In summary, single crystals of PHA, a prototypic class I TS material [10] , exhibit a multitude of extraordinary phenomena. The impressive crystal motility is instigated by a first-order TS phase transition in the TS phase (α), preceded by a colossal expansion along the a axis, strong expansion along the b axis and negative expansion along the c axis. On a molecular scale, the TS transition is due to small, displacive, diffusionless and distortive structural perturbation, where the PHA molecules slide atop each other. The internal strain that develops in response to the strong thermal anisotropy drives two phase transitions above and two phase transitions below ambient temperature. Comparison of the thermodynamic, mechanochemical and kinetic profiles of TS and non-TS transitions between the five polymorphs points out to several requirements for the TS effect. The TS-active structure (α) is soft and remarkably susceptible to internal strain. In a heated, non-pressed crystal, accumulation of strain above a threshold triggers a rapid, self-perpetuated transformation of 10 9 molecules per second with a front of the new phase that on average propagates at speed of 0.54 m s –1 throughout the crystal, ~10 4 times faster than that of the non-TS transition and the more common spin-crossover transitions. This rapid progression causes sudden expansion along the longest axis of the crystal, whereby the crystal is fiercely propelled. The collection of properties of the TS transitions is qualitatively consistent with those observed in inorganic martensites, in support of the hypothesis that these self-actuated materials can be considered organic-based martensites. Synthesis and characterization Complete details of the experimental and theoretical procedures are deposited as Supplementary Methods . PHA was prepared according to a previously published procedure [17] and recrystallized by slow evaporation from toluene or butyronitrile or by sublimation. DSC analysis of PHA samples was carried out on TA DSC-Q2000 instrument by using ca . 2–4 mg of the samples and empty T zero aluminium pan as reference. In a typical measurement, the samples were taken on a T zero aluminium pan and heated from RT (300.6 K) to the selected temperature at a heating rate of 10 K min –1 . The ultraviolet-visible spectra were recorded at RT in absorption mode with Shimadzu UV-3600 UV–vis-NIR spectrometer. The single-crystal XRD data were collected with a Bruker APEX DUO [25] diffractometer using monochromated Mo K α radiation ( λ =0.71069 Å) and CCD as area detector ( Supplementary Data 1 ). For refinement of the crystal structures of ε and γ, high-resolution diffraction data were collected at 365 and 90 K at the ID31 High-Resolution Powder Diffraction Beamline of the European Synchrotron Radiation Facility with wavelength of 0.40000(1) Å, using a nine-stage crystal analyser detector. For studying the thermal expansion, XRPD patterns were collected with a laboratory powder diffractometer Stoe Stadi-P using Cu K α 1 radiation from primary Ge(111)-Johannson-type monochromator and Dectris-MYTHEN 1K strip PSD with an opening angle of 12° in 2 θ , in Debye–Scherrer geometry. Theoretical calculations of the compounds were performed using DFT on GAUSSIAN 09 programme [26] . The 6–311G* basis sets and the LANL2DZ basis set were used for lighter atoms and palladium atoms, respectively. Accession codes: The X-ray crystallographic coordinates for structures reported in this article have been deposited at the Cambridge Crystallographic Data Centre (CCDC), under deposition number CCDC 1013645–1013657. These data can be obtained free of charge from The CCDC via http://www.ccdc.cam.ac.uk/data_request/cif How to cite this article: Panda, M. K. et al. Colossal positive and negative thermal expansion and thermosalient effect in a pentamorphic organometallic martensite. Nat. Commun. 5:4811 doi: 10.1038/ncomms5811 (2014).